Sensing of mammalian IL-17A regulates fungal adaptation and virulence Infections by opportunistic fungi have traditionally been viewed as the gross result of a pathogenic automatism, which makes a weakened host more vulnerable to microbial insults. However, fungal sensing of a host's immune environment might render this process more elaborate than previously appreciated. Here we show that interleukin (IL)-17A binds fungal cells, thus tackling both sides of the host–pathogen interaction in experimental settings of host colonization and/or chronic infection. Global transcriptional profiling reveals that IL-17A induces artificial nutrient starvation conditions in Candida albicans , resulting in a downregulation of the target of rapamycin signalling pathway and in an increase in autophagic responses and intracellular cAMP. The augmented adhesion and filamentous growth, also observed with Aspergillus fumigatus , eventually translates into enhanced biofilm formation and resistance to local antifungal defenses. This might exemplify a mechanism whereby fungi have evolved a means of sensing host immunity to ensure their own persistence in an immunologically dynamic environment. Commensal organisms and mammalian immune mechanisms continuously exchange information, and microbes have developed a contingency-based system during coevolution to guarantee their own persistence in a host by balancing the costs and benefits of expressing virulence. This implies considerable flexibility in virulence manifestation—not to terminate an ongoing symbiosis—and a potential for plasticity in gene expression in response to changes in the host, including the development of acquired immunity. As a consequence, microbes must possess specialized systems that sense and promptly respond to immune activation. Recent progress in our understanding of how fungal signalling circuits operate at the molecular level in sensing environmental factors suggests that this process is much more complex than previously appreciated [1] , [2] . The diploid opportunistic fungal pathogen Candida albicans is a commensal of human mucosal surfaces. Candida infections have typically been thought to rely on an increased susceptibility of weakened hosts to microbial virulence mechanisms. In the case of C. albicans , the increased susceptibility to infection is reflected by fungal transition from a symbiotic to pathogen phenotype. This involves an ability to sense complex environmental signals as well as undergo changes in morphology and virulence [3] . Genome-wide expression profiling has revealed that the initial contact with the host as well as disease progression is associated with changes in transcriptional expression of C. albicans genes that control metabolic and stress adaptation responses. These adaptive responses occur in a niche-specific fashion [2] . Several components of the Candida cell wall have been identified that are capable of binding host proteins and will, at the same time, affect growth, morphogenesis and virulence of the fungus [4] , [5] , [6] . In line with what is observed in humans [7] , Candida overgrowth occurs under conditions of defective interleukin (IL)-17F [8] or IL-17RA signalling [8] , [9] , [10] , which suggests the importance of IL-17RA signalling in preventing infection. Under specific circumstances, IL-17A may, in fact, contribute to disease susceptibility in a host-autonomous fashion, perhaps by modifying the intrinsic virulence of the fungus [8] . In this study, we provide molecular evidence that fungal pathogens may exploit, via a conserved family of glycosylphosphatidylinositol (GPI)-anchored crosslinking proteins, host immunity mediators—specifically, IL-17A—for adaptation, not necessarily implicating virulence, and pathogenesis in mammalian hosts. IL-17A promotes fungal aggregation and filamentation We studied any possible direct effects of IL-17A on C. albicans. We cultured Candida cells in an amino-acid-rich liquid medium (RPMI-1640), which is generally considered to be a physiologically relevant environment [11] —at 37 °C for 24 h or under conditions of biofilm formation. IL-17A was added at concentrations of 1 or 10 ng ml −1 , and cells were examined by light or scanning electron microscopy (SEM) ( Supplementary Methods ) at different times. IL-17A increased cell aggregation at 4 h ( Fig. 1a ) and germination at 24 h ( Fig. 1b ) in a dose-dependent fashion. The percentage of germinated cells was not increased at 4 h, a time when only 10–15% of the treated cells had germinated, as opposed to >40% germinated, control cells ( Fig. 1c ). IL-17A also enhanced biofilm formation, as proven by profuse growth and dense aggregation on SEM examination ( Fig. 1d,e ). IL-17A-treated cells were metabolically active, as shown by viable cell counts ( Fig. 1f ) and staining profiles with a fluorescent probe (FUN-1; Fig. 1g–l ) ( Supplementary Methods ). By epifluorescence microscopy (590-nm excitation; 610-nm emission), C. albicans cells treated with IL-17A and stained with FUN-1 manifested bright red–orange fluorescent structures that correlated with fungal metabolic activity and viability. FUN-1 staining also indicated the presence of true hyphae. 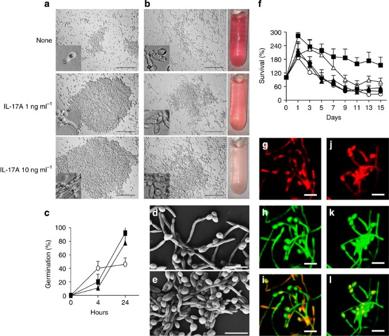Figure 1: IL-17A promotes cellular aggregation and filamentation inC. albicans. Dose-dependent increase ofC. albicans(SC5314) aggregation after 4-h exposure (a) and filamentation after 24-h exposure (b) to different concentrations of IL-17A in RPMI-1640 liquid medium. Cells aliquots were imaged by microscopy and magnified in the insets. Also note the increased turbidity of cell suspension at 24 h. Scale bars, 100 μm. (c) Percentages of germination ofC. albicansuntreated (vehicle-treated, open circle) or treated with IL-17A at 1 (black triangle) or 10 ng ml−1(black square) for 4 or 24 h. Data are mean±s.d.P< 0.05, IL-17A-treated versus vehicle-treated cells, at 4 h;P< 0.01 (1 ng) andP< 0.001 (10 ng) at 24 h (one-way analysis of variance Bonferroni post-test) (n=3). (d,e) IL-17A promotes biofilm formation. SEM images ofC. albicansSC5314 untreated (d) or exposed to 10 ng ml−1IL-17A (e) for 4 h and subsequently cultured onto plastic discs for 24 h. Scale bars, 10 μm. (f) IL-17A increases resistance to nitrogen starvation. Cells were first grown in YPD medium overnight and then switched to nitrogen-free SLAD medium in the presence of 10 ng ml−1IL-17A. Viability, expressed as a percentage of colony-forming units at zero time, was measured over a 15-day period. Cells were exposed to 0.1 (black circle), 1 (black triangle) or 10 ng ml−1(black square) IL-17A or drug vehicle (open circle) at the beginning of the cultures or, in the case of 1 ng ml−1(open triangle), also added every two other days. Data are mean±s.d.P-values ranged from <0.05 to <0.001 for all samples treated with 10 ng IL-17A;P<0.05, on days 3 and 5 for samples treated 1 ng IL-17A every two other days (one-way analysis of variance Bonferroni post-test) (n=3). (g,l)C. albicanscells are metabolically active. Untreated (g–i) or IL-17A-treated (10 ng ml−1in RPMI-1640 liquid media for 24 h) (j–l) cells were red after staining with FUN-1 (g,j), green with Con A (h,k) and yellow in the merged images (i,l). Metabolically active cells are shown in red, and cell wall polysaccharides are shown in green. Scale bars, 5 μm. Images from one representative experiment out of two are shown. Figure 1: IL-17A promotes cellular aggregation and filamentation in C. albicans . Dose-dependent increase of C. albicans (SC5314) aggregation after 4-h exposure ( a ) and filamentation after 24-h exposure ( b ) to different concentrations of IL-17A in RPMI-1640 liquid medium. Cells aliquots were imaged by microscopy and magnified in the insets. Also note the increased turbidity of cell suspension at 24 h. Scale bars, 100 μm. ( c ) Percentages of germination of C. albicans untreated (vehicle-treated, open circle) or treated with IL-17A at 1 (black triangle) or 10 ng ml −1 (black square) for 4 or 24 h. Data are mean±s.d. P < 0.05, IL-17A-treated versus vehicle-treated cells, at 4 h; P < 0.01 (1 ng) and P < 0.001 (10 ng) at 24 h (one-way analysis of variance Bonferroni post-test) ( n= 3). ( d , e ) IL-17A promotes biofilm formation. SEM images of C. albicans SC5314 untreated ( d ) or exposed to 10 ng ml −1 IL-17A ( e ) for 4 h and subsequently cultured onto plastic discs for 24 h. Scale bars, 10 μm. ( f ) IL-17A increases resistance to nitrogen starvation. Cells were first grown in YPD medium overnight and then switched to nitrogen-free SLAD medium in the presence of 10 ng ml −1 IL-17A. Viability, expressed as a percentage of colony-forming units at zero time, was measured over a 15-day period. Cells were exposed to 0.1 (black circle), 1 (black triangle) or 10 ng ml −1 (black square) IL-17A or drug vehicle (open circle) at the beginning of the cultures or, in the case of 1 ng ml −1 (open triangle), also added every two other days. Data are mean±s.d. P -values ranged from <0.05 to <0.001 for all samples treated with 10 ng IL-17A; P <0.05, on days 3 and 5 for samples treated 1 ng IL-17A every two other days (one-way analysis of variance Bonferroni post-test) ( n= 3). ( g , l ) C. albicans cells are metabolically active. Untreated ( g – i ) or IL-17A-treated (10 ng ml −1 in RPMI-1640 liquid media for 24 h) ( j – l ) cells were red after staining with FUN-1 ( g , j ), green with Con A ( h , k ) and yellow in the merged images ( i , l ). Metabolically active cells are shown in red, and cell wall polysaccharides are shown in green. Scale bars, 5 μm. Images from one representative experiment out of two are shown. Full size image Morphological transition in Candida occurs in response to a variety of environmental factors, including amino-acid availability and pH changes [2] , [12] , [13] . To determine whether the effects of IL-17A on the fungus were unique to specific experimental settings, cells were exposed to IL-17A under conditions of limited (SPIDER medium) or rich (YPD medium) nutrient availability, nitrogen starvation (SLAD medium) or alkaline pH (M199 medium), in liquid or solid cultures. IL-17A increased cellular aggregation in SPIDER, SLAD and M199 but not in YPD media ( Supplementary Fig. S1a ). IL-17A also promoted filamentation in SPIDER and M199 media under liquid ( Supplementary Fig. S1b ) or solid ( Supplementary Fig. S1c ) culture conditions, suggesting that IL-17A may exploit pathways of cellular aggregation and filamentation under permissive conditions. The lack of filamentation observed in SLAD medium might indicate that aggregation and filamentation occur independently of each other. To determine whether other cytokines could mimic the effects of IL-17A, we exposed C. albicans to murine IL-17F, IL-17A/IL-17F heterodimer, IL-17E, IL-12p70, IL-23, interferon (IFN)-γ, IL-4 or IL-10. Of these cytokines, only IL-17F and the IL-17A/IL-17F replicated the effects of IL-17A ( Supplementary Fig. S1d ). Consistent with previous data [14] , germination was inhibited by IFN-γ, an effect opposed by the co-presence of IL-17A, both in vitro ( Supplementary Fig. S1d ) and in vivo in C. albicans infection ( Supplementary Fig. S1e–h ). Thus, IL-17A at concentrations encompassing or exceeding those measured in infected organs of wild-type and, particularly, IL-17F-deficient mice ( Supplementary Fig. S2a–i ) may affect fungal growth and morphology. However, owing to rapid degradation, the concentrations of IL-17A measured in ex vivo samples might be considerably lower than those in actual tissue microenvironments [15] . IL-17A affects the transcriptional profile of C. albicans We focused on potential signalling events triggered by IL-17A in C. albicans . We examined the genome-wide transcriptional profile of the fungus exposed to 10 ng ml −1 IL-17A for 4 or 24 h at 37 °C in RPMI-1640 liquid medium. Gene expression analysis indicated that more than 60 transcripts were affected by short-term (4 h) exposure to IL-17A ( Fig. 2a ). Of these, 40 genes encoding components of the translational machinery were downregulated transcriptionally ( Supplementary Data 1 ). Downregulated genes related to ribosome biogenesis, permease/transporter functions, filamentous growth, meiosis, rRNA-processing enzymes, transcription, glycolysis and protein synthesis. At the same time, short-term exposure to IL-17A doubled the expression of 21 genes ( Fig. 2a ). Among those were genes involved in autophagy, a major eukaryotic process by which bulk cytoplasmic components are degraded in the vacuole/lysosome in response to starvation ( Fig. 2b and Supplementary Data 1 ). Those genes included RIC1 , which is related to intracellular trafficking [16] and proteins of the vacuolar protein sorting (Vps) system, such as the Candida orthologue ( orf. 19.130 ) of the serine/threonine protein kinase Vps15. Vps15 has a role in yeast autophagy in response to nutrient starvation [17] , and functions as a membrane-associated complex with class III phosphoinositide 3-kinase [17] , [18] . Overall, the IL-17A-modulated transcriptional profile mirrored that induced in C . albicans by rapamycin [4] , suggesting a role for inhibition of the target of rapamycin (TOR) signalling pathway in the activation of autophagy by IL-17A. Consistently, the TOR inhibitor LPF18 and the downstream orf. 19.4325 gene—an orthologue of Saccharomyces cerevisiae MUC1 coding for an adhesion protein [19] —were upregulated ( Fig. 2c ). 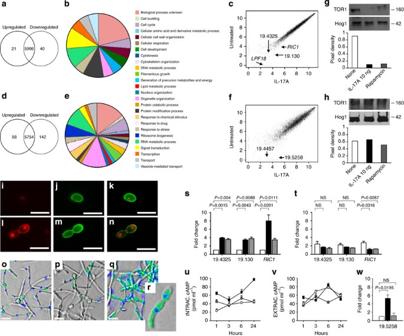Figure 2: Transcriptional profile ofC. albicansin response to IL-17A. (a,d)Venn diagram showing up or downregulated genes, (b,e) GO processes of open reading frames, (c,f) histogram of microarray data fromCandidaSC5314 cells exposed to IL-17A (10 ng) for 4 h (a–c) and 24 h (d–f). Text and arrows: genes involved in TOR pathway at 4 h (c) and of hyphae-induced genes at 24 h (f). (g,h) TOR inhibition in cells treated with 10 ng ml−1IL-17A, 15 nM rapamycin or vehicle (none) by western blotting after 4-h (g) or 24-h (h) exposure. (i–n) Immunofluorescence of ATG8 in untreated (i–k) or IL-17A-treated (10 ng ml−1for 4 h) (l–n) cells. Cells were red after TRITC–ATG8 staining (i,l), green after ConA staining (j,m), merged images (k,n). Mean values (% ATG8+cells (merge); mean±s.d.): ATG8/none, 8.2±1.6; ATG8/IL-17A, 58.0±11.3 (P=0.002) (n=3). Scale bars, 10 μm. (o–r) Monodansilcadaverine (MDC) labelling performed on cells unexposed (o) or exposed to 1 (p) or 10 ng ml−1(q) IL-17A for 4 h. Cells were magnified in the inset (r). Representative results from three independent experiments. The mean values (% hyphal cells with MDC-stained organelles (merge); mean±s.d.) were as follows: none, 9.5±3.2; 1 ng ml−1IL-17A, 14.0±4.7; 10 ng ml−1IL-17A, 56.2±18.71 (P=0.004, IL-17A 10 ng ml−1versus none). Scale bars, 10 μm. (s,t) Quantitative real-time PCR oforfs.19.4325,19.130,RIC1on cDNA fromCandidaSC5314 (s) or theTOR1-1/TOR1mutant (t) strains exposed to vehicle (open column), 10 ng ml−1IL-17A (black column) or 15 nM rapamycin (grey column) for 4 h. The actualP-values are indicated (two-tailedt-test) (n=3). (u,v) Intracellular (u) or extracellular (v) cAMP levels, vehicle (open circle), 10 ng ml−1IL-17A (black square) or rapamycin (grey square).P<0.05, IL-17A-treated versus untreated at 1 h andP<0.01, IL-17A-treated versus untreated at 24 h (u), andP<0.05, rapamycin-treated versus untreated at 6 h (v) (one-way analysis of variance Bonferroni post-test) (n=3). (w)orf. 19.5258expression after 24-hCandidaSC5314 exposure as in (n,o). Data are mean±s.d. (n=3). The actualP-values are indicated (two-tailedt-test). Figure 2: Transcriptional profile of C. albicans in response to IL-17A. ( a,d )Venn diagram showing up or downregulated genes, ( b , e ) GO processes of open reading frames, ( c , f ) histogram of microarray data from Candida SC5314 cells exposed to IL-17A (10 ng) for 4 h ( a – c ) and 24 h ( d – f ). Text and arrows: genes involved in TOR pathway at 4 h ( c ) and of hyphae-induced genes at 24 h ( f ). ( g , h ) TOR inhibition in cells treated with 10 ng ml −1 IL-17A, 15 nM rapamycin or vehicle (none) by western blotting after 4-h ( g ) or 24-h ( h ) exposure. ( i – n ) Immunofluorescence of ATG8 in untreated ( i – k ) or IL-17A-treated (10 ng ml −1 for 4 h) ( l – n ) cells. Cells were red after TRITC–ATG8 staining ( i , l ), green after ConA staining ( j , m ), merged images ( k , n ). Mean values (% ATG8 + cells (merge); mean±s.d. ): ATG8/none, 8.2±1.6; ATG8/IL-17A, 58.0±11.3 ( P =0.002) ( n= 3). Scale bars, 10 μm. ( o – r ) Monodansilcadaverine (MDC) labelling performed on cells unexposed ( o ) or exposed to 1 ( p ) or 10 ng ml −1 ( q ) IL-17A for 4 h. Cells were magnified in the inset ( r ). Representative results from three independent experiments. The mean values (% hyphal cells with MDC-stained organelles (merge); mean±s.d.) were as follows: none, 9.5±3.2; 1 ng ml −1 IL-17A, 14.0±4.7; 10 ng ml −1 IL-17A, 56.2±18.71 ( P =0.004, IL-17A 10 ng ml −1 versus none). Scale bars, 10 μm. ( s , t ) Quantitative real-time PCR of orfs . 19.4325 , 19.130 , RIC1 on cDNA from Candida SC5314 ( s ) or the TOR1-1/TOR1 mutant ( t ) strains exposed to vehicle (open column), 10 ng ml −1 IL-17A (black column) or 15 nM rapamycin (grey column) for 4 h. The actual P -values are indicated (two-tailed t -test) ( n =3). ( u , v ) Intracellular ( u ) or extracellular ( v ) cAMP levels, vehicle (open circle), 10 ng ml −1 IL-17A (black square) or rapamycin (grey square). P <0.05, IL-17A-treated versus untreated at 1 h and P <0.01, IL-17A-treated versus untreated at 24 h ( u ), and P <0.05, rapamycin-treated versus untreated at 6 h ( v ) (one-way analysis of variance Bonferroni post-test) ( n= 3). ( w ) orf. 19.5258 expression after 24-h Candida SC5314 exposure as in ( n , o ). Data are mean±s.d. ( n =3). The actual P -values are indicated (two-tailed t -test). Full size image Although the patterns observed for some genes at 4 h occasionally persisted over time (such as the upregulation of MUC1 ), the transcriptional profile observed after prolonged exposure to IL-17A was considerably different. Candida exposure to the cytokine for 24 h resulted in the induction of 58 genes ( Fig. 2d ) involved in cell mitosis, ribosome biogenesis, transcription and cell wall remodelling ( Fig. 2e and Supplementary Data 1 ). Of interest, classic hyphae-induced genes were increased in expression, such as BNI4 ( orf 19.4457 ) [20] and an orthologue of S. cerevisiae adenylate cyclase Cyr1 ( orf. 19.5258 ) ( Fig. 2f ). Cyr1p is a key component of the cAMP/PKA signaling pathway directly involved in signal sensing and in controlling hyphal morphogenesis in C. albicans [21] . To substantiate the global transcriptional profiling data, we performed western blotting, fluorescence microscopy, real-time quantitative reverse transcriptase PCR and enzyme-linked immunosorbent assays to measure the levels of proteins or monitor functions associated with the differentially regulated genes (that is, TOR1, autophagy and extracellular/intracellular cAMP). Similar to the effect of rapamycin, TOR1 expression was reduced after 4 h ( Fig. 2g ) but not 24-h ( Fig. 2h ) exposure to IL-17A and, accordingly, autophagy was induced, as revealed by ATG8 immunofluorescence ( Fig. 2i–n ), monodansilcadaverine (MDC) labelling ( Fig. 2o–r ) and increased expression of the autophagy-related genes ( Fig. 2s ). We used the C. albicans TOR1-1/TOR1 mutant [4] to evaluate the role of the TOR pathway in IL-17A signalling. We found that the effects of IL-17A on autophagy-related gene expression ( Fig. 2t ) and cell aggregation ( Supplementary Fig. S3a–d ) could not be observed in this mutant. At variance with rapamycin, intracellular cAMP levels ( Fig. 2u,v ) and expression of the Cyr1 orthologue gene ( Fig. 2w ) were increased after 24-h exposure to IL-17A. Thus, although autophagic flux was not measured, the data suggest that the TOR pathway mediates autophagy and cell aggregation in response to IL-17A but is dispensable for hyphal induction. In fact, filamentation of the TOR1-1/TOR1 mutant was observed after exposure to IL-17A ( Supplementary Fig. S3c,d ). IL-17A binds C. albicans C. albicans binds a variety of host proteins that affect fungal morphology and virulence [4] , [6] . We examined whether IL-17A directly binds the fungus in vitro . An indirect immunofluorescence assay revealed the presence of Candida cells with bound IL-17A. Binding was affected significantly by growth phase of the fungus, as intense binding was observed on hyphal tips and not on parent blastospores ( Fig. 3a–g ). Not all hyphal tips stained with the same intensity. Thus, IL-17A binds C. albicans components expressed during hyphal growth. To assess whether ex vivo Candida cells also bind IL-17A, we used C. albicans isolates freshly obtained from different human anatomical sites. All of the analysed C . albicans isolates, and particularly those from the gut and vagina, were able to bind murine ( Fig. 3h ) and human ( Fig. 3i ) IL-17A. Notably, freshly isolated samples from vaginal fluids stained positive with an anti-IL-17A antibody ( Fig. 3j–o ), suggesting that binding to IL-17A may occur in vivo at the infected sites. Levels of IL-17A in human vaginal fluids ranged from 80 to 240 pg ml −1 . Murine studies confirmed that IL-17A may bind to the fungus in the vagina as revealed by the presence of numerous hyphae in the vagina of IL-17F-deficient (that is, in conditions of high levels of IL-17A) but not IL-17A-deficient or wild-type mice intravaginally injected with C. albicans blastospores ( Fig. 3p–r ). Binding was also observed, albeit to a lesser extent, with other yeast species, such as C. glabrata , C . krusei and S. cerevisiae ( Fig. 3s ). 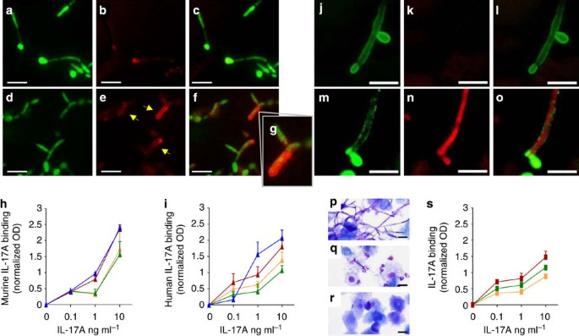Figure 3: IL-17A bindsC. albicans. (a–g) GFPC. albicanscells were untreated (a–c) or treated (d–g) for 4 h with 10 ng ml−1IL-17A followed by anti-IL17A-PE and examined by fluorescence microscopy (scale bars, 5 μm). Cells were green in (a,d), red upon staining with anti-IL17A-PE (b,e) and double stained in the merged images (c,f). Note the binding of IL-17A to hyphal tips (arrows and magnified ing) (n=3). Images are from one representative experiment out of three. (h,i) Binding of murine (h) or human (i) IL-17A to clinical isolates ofC. albicansfrom human urine (yellow triangle), blood (green triangle), vagina (red triangle) and gut (blue triangle). IL-17A was added to paraformaldehyde-fixed fungal cells followed by biotinylated secondary anti-IL-17A antibody and streptavidin-horse radish peroxidase. The optical density at 450 nm was corrected by subtracting the optical density at 570 nm (normalized OD) in the enzyme-linked immunosorbent assay.P-values of samples exposed to 0.1 and 1 ng IL-17A ranged from <0.05 to <0.001 (one-way analysis of variance Bonferroni post-test). All samples exposed to 10 ng IL-17A displayed significant (P<0.001, one-way analysis of variance Bonferroni post-test) OD values relative to unexposed samples (0). (j–o) Direct visualization of IL-17A onCandidafreshly harvested from human vagina. Same experiment as in (a–g) on cells previously stained with Con A (j,m, green) and incubated with PE-anti-human IL-17A (k,n, red) and double stained in the merged images (l,o). Scale bars, 10 μm. Shown is one representative experiment out of three. (p–r) Cytospins of vaginal fluids from IL-17F-deficient (p), IL-17A-deficient (q) and C57BL/6 (r) mice intravaginally infected two days before withC.albicansSC5314 blastospores. Note the presence of hyphae in the vagina of IL-17F-deficient mice after May–Grünwald–Giemsa staining (scale bars, 20 μm). Shown is one representative experiment out of three. (s) Binding of IL-17A to clinical isolates ofC. krusei(red square),C. glabrata (green square) andS. cerevisiae(yellow square) done as in (h,i). All samples exposed to IL-17A displayed significant (P<0.001, one-way analysis of variance Bonferroni post-test) OD values (n=3). Data are mean±s.d. (n=4). Figure 3: IL-17A binds C. albicans . ( a – g ) GFP C. albicans cells were untreated ( a – c ) or treated ( d – g ) for 4 h with 10 ng ml −1 IL-17A followed by anti-IL17A-PE and examined by fluorescence microscopy (scale bars, 5 μm). Cells were green in ( a , d ), red upon staining with anti-IL17A-PE ( b , e ) and double stained in the merged images ( c , f ). Note the binding of IL-17A to hyphal tips (arrows and magnified in g ) ( n =3). Images are from one representative experiment out of three. ( h , i ) Binding of murine ( h ) or human ( i ) IL-17A to clinical isolates of C. albicans from human urine (yellow triangle), blood (green triangle), vagina (red triangle) and gut (blue triangle). IL-17A was added to paraformaldehyde-fixed fungal cells followed by biotinylated secondary anti-IL-17A antibody and streptavidin-horse radish peroxidase. The optical density at 450 nm was corrected by subtracting the optical density at 570 nm (normalized OD) in the enzyme-linked immunosorbent assay. P -values of samples exposed to 0.1 and 1 ng IL-17A ranged from <0.05 to <0.001 (one-way analysis of variance Bonferroni post-test). All samples exposed to 10 ng IL-17A displayed significant ( P <0.001, one-way analysis of variance Bonferroni post-test) OD values relative to unexposed samples (0). ( j – o ) Direct visualization of IL-17A on Candida freshly harvested from human vagina. Same experiment as in ( a – g ) on cells previously stained with Con A ( j , m , green) and incubated with PE-anti-human IL-17A ( k , n , red) and double stained in the merged images ( l , o ). Scale bars, 10 μm. Shown is one representative experiment out of three. ( p–r ) Cytospins of vaginal fluids from IL-17F-deficient ( p ), IL-17A-deficient ( q ) and C57BL/6 ( r ) mice intravaginally infected two days before with C.albicans SC5314 blastospores. Note the presence of hyphae in the vagina of IL-17F-deficient mice after May–Grünwald–Giemsa staining (scale bars, 20 μm). Shown is one representative experiment out of three. ( s ) Binding of IL-17A to clinical isolates of C. krusei (red square), C. glabrata ( green square) and S. cerevisiae (yellow square) done as in ( h , i ). All samples exposed to IL-17A displayed significant ( P <0.001, one-way analysis of variance Bonferroni post-test) OD values ( n =3). Data are mean±s.d. ( n =4). Full size image IL-17A binds GPI-anchored fungal proteins To identify the putative fungal ligand(s) involved in IL-17A effects, we studied binding of IL-17A to purified proteins and polysaccharides from the fungal cell wall. IL-17A selectively bound members of the Crh and Gas GPI-anchored protein family, namely Crh11p and Gas1p, and did not bind fungal polysaccharides ( Fig. 4a ). No binding was observed with IL-17E ( Fig. 4a ) or other cytokines (data not shown). Anti-IL-17A or anti-Crh11p antibody inhibited binding ( Supplementary Fig. S4a ), and Crh11p inhibited binding of IL-17A to whole fixed hyphae ( Supplementary Fig. S4b ). A strong protein-to-protein interaction was observed in co-immunoprecipitation experiments with anti-IL-17A and anti-Crh11p ( Fig. 4b ). These data suggested that fungal Crh11p might act as a binding structure (that is, an acceptor rather than a signalling receptor) for host-derived IL-17A. Notably, IL-17A failed to bind mutant Candida strains in which all three genes of the CRH family (namely, UTR2 , CRH11 and CRH12) had been deleted [22] , yet binding was restored by CRH11 or CRH12 reconstitution ( Fig. 4c ). Consistent with the notion that Crh11p, more than Crh12p, is cell cycle regulated and expressed under sporulation conditions [23] , of the two mutant strains, crh11 Δ but not crh12 Δ failed to respond to IL-17A with adhesion and filamentation ( Supplementary Fig. S4c,d ) ( Supplementary Methods ) as well as with internalization of bound IL-17A ( Fig. 4d,e ). Thus, IL-17A binds different members of the CRH family in Candida , and, specifically, Crh11p appears to be necessary for IL-17A effects on the fungus. 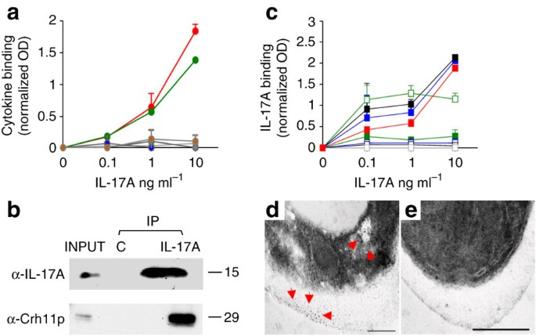Figure 4: IL-17A binds Crh11p of theCandidaCRH family. (a) Dose-dependent binding of IL-17A to fungal Crh11p (red circle) and Gas1p (light blue circle) proteins, but not to the fungal polysaccharides β-1,3-D-glucan (open circle), mannan (blue circle) and zymosan (grey circle). The lack of binding of IL-17E to Crh11p (orange circle) serves as a negative control. The optical density at 450 nm was corrected by subtracting the optical density at 570 nm (normalized OD) in the enzyme-linked immunosorbent assay. Data are mean±s.d.,n=3.P<0.001, Crh11p and Gas1p without versus with IL-17A (one-way analysis of variance Bonferroni post-test). (b) Co-immunoprecipitation assay of fungal Crh11p and murine IL-17A proteins. Immunoprecipitates were probed with antibodies to the corresponding antigens and secondary HRP-conjugated antibody. C, irrelevant antibody. (c) Failure of IL-17A to bind to wild-type (red square) or mutantC. albicansstrains in which the three genes of the CRH family (UTR2,open light blue,CRH1, open black and CRH12, open blue square) had been deleted, and restoration of binding byCRH1(black square) andCRH12(blue square), but notUTR2(light blue square), reconstitution. Data are mean±s.d. (n=3).P<0.001 for red square, open light blue, black square and blue square (one-way analysis of variance Bonferroni post-test). (d,e) Cellular localization of bound IL-17A. Electron micrographs of ultrafine sections ofC. albicansMKY 378 wild-type (d) or thecrh11Δ mutant (e) incubated with biotinylated IL-17A and streptavidin gold-conjugated particles. Arrows indicate immunogold particles. Scale bars, 200 nm. Figure 4: IL-17A binds Crh11p of the Candida CRH family. ( a ) Dose-dependent binding of IL-17A to fungal Crh11p (red circle) and Gas1p (light blue circle) proteins, but not to the fungal polysaccharides β-1,3- D -glucan (open circle), mannan (blue circle) and zymosan (grey circle). The lack of binding of IL-17E to Crh11p (orange circle) serves as a negative control. The optical density at 450 nm was corrected by subtracting the optical density at 570 nm (normalized OD) in the enzyme-linked immunosorbent assay. Data are mean±s.d., n =3. P <0.001, Crh11p and Gas1p without versus with IL-17A (one-way analysis of variance Bonferroni post-test). ( b ) Co-immunoprecipitation assay of fungal Crh11p and murine IL-17A proteins. Immunoprecipitates were probed with antibodies to the corresponding antigens and secondary HRP-conjugated antibody. C, irrelevant antibody. ( c ) Failure of IL-17A to bind to wild-type (red square) or mutant C. albicans strains in which the three genes of the CRH family ( UTR2, open light blue, CRH1 , open black and C RH12 , open blue square) had been deleted, and restoration of binding by CRH1 (black square) and CRH12 (blue square), but not UTR2 (light blue square), reconstitution. Data are mean±s.d. ( n =3). P <0.001 for red square, open light blue, black square and blue square (one-way analysis of variance Bonferroni post-test). ( d , e ) Cellular localization of bound IL-17A. Electron micrographs of ultrafine sections of C. albicans MKY 378 wild-type ( d ) or the crh11 Δ mutant ( e ) incubated with biotinylated IL-17A and streptavidin gold-conjugated particles. Arrows indicate immunogold particles. Scale bars, 200 nm. Full size image IL-17A sensing in vivo As both adhesion and hyphal growth are considered to be important for pathogenicity [24] , we assessed whether the increased fungal adhesion and filamentation induced by IL-17A might have biological relevance in vivo . For this purpose, we evaluated whether binding to IL-17A could be demonstrated on fungi in vivo , the consequences in terms of fungal growth and morphology, and the involvement of the CRH family proteins. We found that IL-17A bound the fungus in the stomachs of wild-type ( Fig. 5a–c ), IL-17F-deficient ( Fig. 5d–f ) but not IL-17A-deficient ( Fig. 5g–i ) mice intragastrically infected with the fungus, and this was associated with germination in wild-type mice ( Fig. 5j ), hyphal formation in IL-17F-deficient mice ( Fig. 5k ) and neither one in IL-17A-deficient mice ( Fig. 5l ). Thus, despite the ability of IL-17F to mimic IL-17A effects in vitro ( Supplementary Fig. S1d ), a lower production of IL-17F in vivo ( Supplementary Fig. S2g–i ) might account for the lack of IL-17F activity on the fungus at sites of infection. We also evaluated the effects of pre-exposure of C. albicans to IL-17A in vitro on fungal growth and virulence in the orogastric as well as the oropharyngeal models of candidiasis. We found that IL-17A-treated Candida cells were more virulent in vivo , as indicated by increased fungal load ( Fig. 5m ) and local inflammatory pathology in the stomachs of intragastrically infected mice ( Supplementary Fig. S5a,b ). Consistent with the in vitro data, the crh11 Δ, but not the crh12 Δ, mutant was less virulent in vivo and failed to respond to IL-17A with increased virulence ( Fig. 5n,o and Supplementary Fig. S5c–f ). Similar results were obtained in the oropharyngeal model of candidiasis ( Supplementary Fig. S5g–r ). Thus, fungal sensing of IL-17A occurs in vivo via Crh1p, and affects fungal growth and morphology. 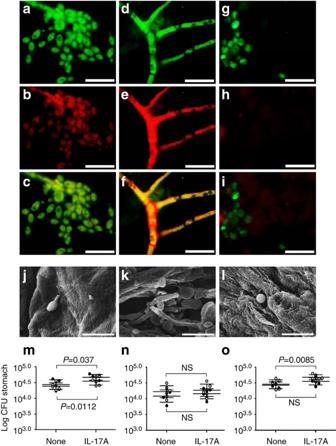Figure 5: IL-17A bindsC. albicans in vivovia Crh11p. Fungi were harvested from the stomachs of C57BL/6 (a–c), IL-17F-deficient (d–f) or IL-17A-deficient (g–i) mice infected with GFP–Candidafor 2 days, and stained using PE-labeled antibody to IL-17A. Cells were green in (a,dandg), red upon staining with anti-IL17A-PE (b,eandh) and double stained in the merged images (c,fandi). Scale bars, 10 μm. Images are from one representative experiment out of two. (j–l) SEM images showing fungal germination in the stomachs of C57BL/6 mice (j), filamentation in IL-17F-deficient mice (k) and neither one in IL-17A-deficient (l) mice intragastrically infected 2 days before. Scale bars, 10 μm. (a–l) Images are from one representative experiment out of two. (m–o) C57BL/6 mice were infected intragastrically withC. albicansMKY 378 strain (m) or thecrh11Δ (n) andcrh12Δ (o) mutants, and were monitored for fungal growth (log10colony-forming units (CFU) at 2 (open circle) or 8 (black circle) days post infection). Data are mean±s.d. (n=3). The actualP-values are indicated (two-tailedt-test) for 2 and 8 days (m) and for 2 days (o). Fungal cells were untreated (none) or exposed to 10 ng ml−1IL-17A for 4 h before injection. Figure 5: IL-17A binds C. albicans in vivo via Crh11p. Fungi were harvested from the stomachs of C57BL/6 ( a – c ), IL-17F-deficient ( d – f ) or IL-17A-deficient ( g – i ) mice infected with GFP– Candida for 2 days, and stained using PE-labeled antibody to IL-17A. Cells were green in ( a , d and g ), red upon staining with anti-IL17A-PE ( b , e and h ) and double stained in the merged images ( c , f and i ). Scale bars, 10 μm. Images are from one representative experiment out of two. ( j–l ) SEM images showing fungal germination in the stomachs of C57BL/6 mice ( j ), filamentation in IL-17F-deficient mice ( k ) and neither one in IL-17A-deficient ( l ) mice intragastrically infected 2 days before. Scale bars, 10 μm. ( a–l ) Images are from one representative experiment out of two. ( m – o ) C57BL/6 mice were infected intragastrically with C. albicans MKY 378 strain ( m ) or the crh11 Δ ( n ) and crh12 Δ ( o ) mutants, and were monitored for fungal growth (log 10 colony-forming units (CFU) at 2 (open circle) or 8 (black circle) days post infection). Data are mean±s.d. ( n =3). The actual P -values are indicated (two-tailed t -test) for 2 and 8 days ( m ) and for 2 days ( o ). Fungal cells were untreated (none) or exposed to 10 ng ml −1 IL-17A for 4 h before injection. Full size image IL-17A induces fungal autophagy in vivo In searching for an explanation for the increased fungal outgrowth, we determined whether IL-17A would favour fungal evasion by assessing susceptibility to killing by effector phagocytes in vitro . We observed that IL-17A increased fungal adhesion on phagocytes, yet it reduced phagocytosis and susceptibility to killing of C. albicans SC5314 ( Fig. 6a ). Although C. albicans may not depend on autophagy for virulence [25] , [26] , we found that adhesion to phagocytes and susceptibility to killing of the mutant strains TOR1-1/TOR1 ( Fig. 6b ) and the atg9 Δ /atg9 Δ, blocked in autophagy [5] , [26] ( Fig. 6c ), were not similarly affected by IL-17A. Thus, much like in Cryptococcus neoformans [18] , the TOR-dependent autophagy pathway might be involved in virulence in vivo . To clarify this issue, we evaluated whether autophagy could be demonstrated at sites of infection, and the impact on fungal adaptation and virulence. Autophagy ( Fig. 6d–f ) and upregulated expression of autophagy-related genes ( Fig. 6g ) were observed in ex vivo Candida SC5314 cells from IL-17F-deficient but not IL-17A-deficient or wild-type mice. Similar to that observed with the crh11 Δ mutant, a reduced fungal growth and inflammatory pathology were observed with the TOR1-1/TOR1 or the atg9 Δ /atg9 Δ mutant strains but not the wild-type or the atg9 Δ /atg9 Δ+ATG9 revertant strains under conditions of IL-17A production, such as in wild-type ( Fig. 6h and Supplementary Fig. S6a–d ) and IL-17F-deficient mice ( Fig. 6i and Supplementary Fig. S6e–g ), but not in the condition of IL-17A deficiency ( Fig. 6j and Supplementary Fig. S6h–j ). Thus, IL-17A sensing via fungal Crh proteins affects fungal fitness in vivo through adaptation mechanisms involving TOR-dependent autophagy and filamentation. 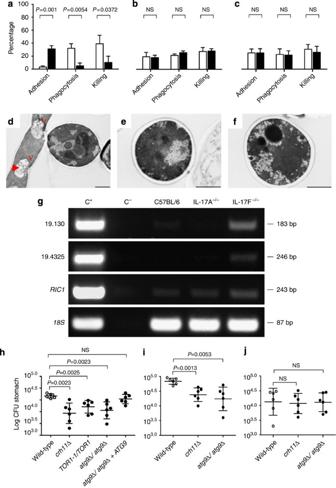Figure 6: IL-17A promotes fungal autophagyin vivo. CandidaSC5314 (a),TOR1-1/TOR1(b) andatg9Δ/atg9Δ (c) mutant strains were untreated (open column) or pre-incubated with IL-17A (filled column) for 4 h before exposure to neutrophils for additional 2 h before the assessment of adhesion, phagocytosis and killing. Error bars, mean±s.d. (n=3). The actualP-values are indicated (two-tailedt-test). (d–f) IL-17A induces autophagyin vivo. Representative electron micrographs of vacuoles (v) inCandidacells purified on sucrose gradient from the stomachs of IL-17F-deficient (d), IL-17A-deficient (e) or C57BL/6 (f) mice intragastrically infected 2 days before. Arrows indicate autophagy-associated structures. Scale bars, 1 μm. (g) Fungi purified from the stomachs of mice infected as in (d–f) were subjected to RT–PCR for autophagy genes expression. C+, fungal cells grown on SPIDER solid medium. C–, no cells. (h–j) Log10colony-forming units (CFU) at 2 days post infection withC. albicansSC5314 (wild-type) or different mutant strains in C57BL/6 (h), IL-17F-deficient (i) or IL-17A-deficient (j) mice. Data are mean±s.d. (n=3). The actualP-values are indicated (two-tailedt-test). Figure 6: IL-17A promotes fungal autophagy in vivo . Candida SC5314 ( a ), TOR1-1/TOR1 ( b ) and atg9 Δ/ atg9 Δ ( c ) mutant strains were untreated (open column) or pre-incubated with IL-17A (filled column) for 4 h before exposure to neutrophils for additional 2 h before the assessment of adhesion, phagocytosis and killing. Error bars, mean±s.d. ( n =3). The actual P -values are indicated (two-tailed t -test). ( d – f ) IL-17A induces autophagy in vivo . Representative electron micrographs of vacuoles (v) in Candida cells purified on sucrose gradient from the stomachs of IL-17F-deficient ( d ), IL-17A-deficient ( e ) or C57BL/6 ( f ) mice intragastrically infected 2 days before. Arrows indicate autophagy-associated structures. Scale bars, 1 μm. ( g ) Fungi purified from the stomachs of mice infected as in ( d – f ) were subjected to RT–PCR for autophagy genes expression. C + , fungal cells grown on SPIDER solid medium. C – , no cells. ( h – j ) Log 10 colony-forming units (CFU) at 2 days post infection with C. albicans SC5314 (wild-type) or different mutant strains in C57BL/6 ( h ), IL-17F-deficient ( i ) or IL-17A-deficient ( j ) mice. Data are mean±s.d. ( n =3). The actual P -values are indicated (two-tailed t -test). Full size image A. fumigatus senses IL-17A To assess whether A. fumigatus —a ubiquitous fungus that, although not a commensal in the strict sense, is nevertheless in continuous contact with the human upper respiratory tract [27] —also senses IL-17A, we performed binding studies and morphological assays in vitro and in vivo . IL-17A strongly bound to the fungus. Binding was dependent on growth phase of the fungus, being undetectable in resting conidia, but intense in swollen conidia ( Fig. 7a–f ). The fungus responded to IL-17A with biofilm formation ( Fig. 7g,h ) and, similar to rapamycin ( Fig. 7i ) with autophagy ( Fig. 7j,k ). As levels of lung IL-17A ranged from 1.5 (wild-type) up to 9 ng ml −1 (IL-17F-deficient mice) during infection, these data suggest that IL-17A can affect Aspergillus morphology in vivo . 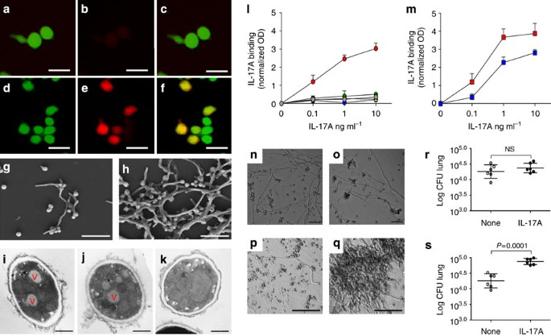Figure 7: IL-17A binds and affects growth and morphology ofA. fumigatus. (a–f) GFPAspergillusconidia, incubated overnight at room temperature, were untreated (a–c) or exposed (d–f) to 10 ng ml−1IL-17A for 4 h followed by anti-IL-17A-PE. Cells were green in (a,b), red upon staining with anti-IL17A-PE (b,e) and double stained in the merged images (c,f). Scale bars, 10 μm. (g,h) IL-17A promotes biofilm formation inA. fumigatusAF293 strain. SEM images refer to cells untreated (g) or pretreated (h) with 10 ng ml−1IL-17A for 4 h and subsequently cultured onto plastic discs for 24 h. Scale bars, 20 μm. (i–k) IL-17A induces autophagy inAspergillus. Representative electron micrographs of vacuoles (v) inA. fumigatusAF293 unexposed (k) or exposed to 10 ng ml−1IL-17A (j) or 15 nM rapamycin (i) for 4 h before TEM. Scale bars, 500 nm. (l) IL-17A binds theAspergillusCrf1p protein. Dose-dependent binding of IL-17A to Crf1p (red circle), Gel1p (light blue circle) or theAspergillus-derived polysaccharides β-1,3-D-glucan (blue circle), α-1,3-D-glucan (open circle) and galactomannan (grey circle). The optical density at 450 nm was corrected by subtracting the optical density at 570 nm (normalized OD) in the enzyme-linked immunosorbent assay (ELISA) on microtitre-coated plates. Data are mean±s.d. (n=5).P-values ranged from <0.01 to 0.001 for IL-17A-treated versus untreated (0) Crf1p (one-way analysis of variance, Bonferroni post-test). (m) ELISA assay showing failure of IL-17A to bind theAspergillusmutantcrf1Δ (blue square) as opposed to the wild-type strain AF293 (red square). Data are mean±s.d. (n=5).P-values ranged from <0.05 to <0.01, wild-type versus mutant strain exposed to 1 or 10 ng ml−1IL-17A (one-way analysis of variance, Bonferroni post-test). (n–q) IL-17A promotes filamentation in the mutantcrf1Δ (o) but not the wild-type AF293 (q) strain after 24-h exposure in liquid culture. Scale bars, 500 μm. (r,s) C57BL/6 mice were infected intranasally with theAspergillus crf1Δ mutant (r) or the AF293 (s) strain and monitored for fungal growth (log10colony-forming units (CFU)±s.d.) in the lungs 2 days later. Fungal cells were exposed or not (none) to 10 ng ml−1IL-17A for 4 h, extensively washed and injected. Data are mean±s.d. (n=4). The actualP-values are indicated (two-tailedt-test). Figure 7: IL-17A binds and affects growth and morphology of A. fumigatus . ( a – f ) GFP Aspergillus conidia, incubated overnight at room temperature, were untreated ( a – c ) or exposed ( d – f ) to 10 ng ml −1 IL-17A for 4 h followed by anti-IL-17A-PE. Cells were green in ( a , b ), red upon staining with anti-IL17A-PE ( b , e ) and double stained in the merged images ( c , f ). Scale bars, 10 μm. ( g , h ) IL-17A promotes biofilm formation in A. fumigatus AF293 strain. SEM images refer to cells untreated ( g ) or pretreated ( h ) with 10 ng ml −1 IL-17A for 4 h and subsequently cultured onto plastic discs for 24 h. Scale bars, 20 μm. ( i – k ) IL-17A induces autophagy in Aspergillus . Representative electron micrographs of vacuoles (v) in A. fumigatus AF293 unexposed ( k ) or exposed to 10 ng ml −1 IL-17A ( j ) or 15 nM rapamycin ( i ) for 4 h before TEM. Scale bars, 500 nm. ( l ) IL-17A binds the Aspergillus Crf1p protein. Dose-dependent binding of IL-17A to Crf1p (red circle), Gel1p (light blue circle) or the Aspergillus -derived polysaccharides β-1,3- D -glucan (blue circle), α-1,3- D -glucan (open circle) and galactomannan (grey circle). The optical density at 450 nm was corrected by subtracting the optical density at 570 nm (normalized OD) in the enzyme-linked immunosorbent assay (ELISA) on microtitre-coated plates. Data are mean±s.d. ( n= 5). P -values ranged from <0.01 to 0.001 for IL-17A-treated versus untreated (0) Crf1p (one-way analysis of variance, Bonferroni post-test). ( m ) ELISA assay showing failure of IL-17A to bind the Aspergillus mutant crf1 Δ (blue square) as opposed to the wild-type strain AF293 (red square). Data are mean±s.d. ( n =5). P -values ranged from <0.05 to <0.01, wild-type versus mutant strain exposed to 1 or 10 ng ml −1 IL-17A (one-way analysis of variance, Bonferroni post-test). ( n – q ) IL-17A promotes filamentation in the mutant crf1 Δ ( o ) but not the wild-type AF293 ( q ) strain after 24-h exposure in liquid culture. Scale bars, 500 μm. ( r , s ) C57BL/6 mice were infected intranasally with the Aspergillus crf1 Δ mutant ( r ) or the AF293 ( s ) strain and monitored for fungal growth (log 10 colony-forming units (CFU)±s.d.) in the lungs 2 days later. Fungal cells were exposed or not (none) to 10 ng ml −1 IL-17A for 4 h, extensively washed and injected. Data are mean±s.d. ( n =4). The actual P -values are indicated (two-tailed t -test). Full size image Orthologues of the GPI CRH family are present in Aspergillus [28] . We assessed whether IL-17A would bind those proteins. Of the two orthologous proteins, Crf1p but not Gel1p bound IL-17A ( Fig. 7l ). As in the Candida setting, no binding was observed to Aspergillus -derived polysaccharides ( Fig. 7l ). IL-17A failed to bind an Aspergillus mutant ( Fig. 7m ) in which the CRF1 gene had been deleted ( Supplementary Fig. S7a,b ). The mutant strain failed to respond to IL-17A in vitro with extensive hyphal growth after 24 h of exposure ( Fig. 7n,o ), as opposed to the wild-type strain ( Fig. 7p,q ). In vivo , the virulence of the mutant strain was not affected upon IL-17A pre-exposure in vitro , as indicated by fungal growth ( Fig. 7r ) and histopathology ( Supplementary Fig. S7c,d ) as opposed to the wild-type strain ( Fig. 7s and Supplementary Fig. S7e,f ). Thus, IL-17A sensing is a feature shared by human commensal and airborne fungi. This study provides molecular evidence that opportunistic pathogens, such as C . albicans and A. fumigatus , may exploit host immunity mediators—specifically, a cytokine—for adaptation to their hosts. Thus, in common with certain opportunistic bacteria—such as Pseudomonas aeruginosa [29] —human fungi might have evolved a contingency-based mechanism to mount an effective countermeasure to immune activation by their host. Although it was previously recognized that IFN-γ inhibits yeast-to-hyphal transition in C. albicans [14] , little progress had been made on the mechanistic details of this early observation. Our data show that a conserved family of GPI-anchored crosslinking enzymes, highly conserved in Candida and Aspergillus , and known to be exposed at growing sites—such as bud emergences or hyphal tips [22] , [23] —and detectable in mice [28] , [30] , [31] as well as in humans [32] , mediates IL-17A sensing by fungi. Thus, in addition to their involvement in adhesion and virulence [6] , [12] , these proteins are immunologically reactive. Intriguingly, our study also suggests that Th1 and Th17 cytokines may have disparate effects on Candida in vitro ( Supplementary Fig. S1d ), as well as in vivo ( Supplementary Fig. S1e–h ), a finding highlighting the complex cross-regulation between Th1 and Th17 responses that would also include an action on fungal cells. Host IL-17A sensing occurs via the TOR nutrient sensing pathway, a conserved mechanism among yeasts and filamentous fungi [33] that regulates autophagy [34] , cell growth and virulence [4] , [18] , [35] . Autophagy is an evolutionary conserved response to stress that has been linked to important protective roles in mammalian cells [36] . In mammalian host–pathogen interactions, the role of autophagy has mostly favoured the host, as induction of autophagy was found to be crucial in the control of some infecting pathogens and in the ensuing immune response [37] , [38] . This study highlights how the TOR nutrient sensing pathway could be exploited by fungi to sense host IL-17A for survival in an immunologically reactive environment, consistent with the view that Th17 immunity develops to maintain mutualism [39] . However, prolonged exposure to IL-17A further affects fungal fitness by inducing filamentation and virulence in a TOR-autonomous fashion. Thus, IL-17A may contribute both to fungal survival, not necessarily implicating virulence, and to pathogenesis in mammalian hosts. Despite a plethora of mechanisms by which autophagy and virulence can be regulated in different fungal infections, our study highlights the unique feature of the amino-acid sensing pathway, a survival strategy under evolutionary pressure [40] , in the interaction of fungi with their mammalian hosts. Strains and growth media A complete list of the strains used in this study is reported in Supplementary Table S1 . C. albicans strains were propagated on Sabouraud's glucose agar 37 °C (Sigma Aldrich, Milan, Italy). Isolation of C. albicans from infected stomachs was done on a sucrose gradient, as described [41] . Viable Aspergillus conidia (>95%) were obtained by growth on potato dextrose agar (PDA) with chloramphenicol 0.05% [w/v], (Difco Laboratories, Detroit, MI, USA) after 4 days at room temperature (RT). Freshly harvested (unpassaged) C. glabrata , C. krusei and S. cerevisiae isolates, obtained from clinical specimens, and C. albicans clinical isolates, derived from blood, urine, vagina and gastrointestinal tract, were kindly provided by the Mycology Section, S. Maria della Misericordia Medical Center, Perugia, Italy. Study approval was provided by the local ethics committee (Umbria Regional Hospital Ethics Committee, CEAS Umbria), and informed written consent was obtained from all participants in accordance with the Declaration of Helsinki. The CAG31A C. albicans mutant strain expressing the GFP gene was obtained as described [42] . When observed by fluorescence microscopy, both yeasts and hyphae of the CAG31A strain were intensively fluorescent [43] . IL-17A binding to fungi by indirect immunofluorescence Localization of IL-17A binding on C. albicans and A. fumigatus was assayed by indirect immunofluorescence using a PE-rat IgG2a raised against mouse IL-17A (clone eBio17B7, e-Bioscience, Prodotti Gianni Milan, Italy). Fungal cells were collected, washed, resuspended in RPMI-1640 medium, placed (1×10 6 cells ml −1 ) on microscope glass slides and incubated overnight at 28 °C for Aspergillus (AF293) and for 4 h at 37 °C for Candida GFP (CAG31A). After adhesion, cell cultures were fixed with 1% formaldehyde. Slides were washed with PBS. Nonspecific binding sites were blocked with PBS/bovine serum albumin (BSA) 2.5% and incubated for 1 h at RT. Cells were incubated with IL-17A (10 ng ml −1 ) for 4 h at RT and then incubated with anti-IL-17A-PE (0.5 μg ml −1 ) in PBS/BSA 2.5% for 1 h at RT. Slides were washed with PBS and mounted on a cover slip with a few drops of Vectashield mounting medium (Vector Laboratories, DBA Italia S.R.L. Milan, Italy). For staining of fungi isolated from the stomachs of Candida GFP-infected mice, tissues were harvested 2 days post infection and processed in RPMI-1640. For staining of Candida from human vaginal fluids, cells recovered after clarifications were stained with Con A-FITC conjugate (25 μg ml −1 ). After blocking of nonspecific binding sites with PBS/BSA 2.5%, the cytospins were incubated for 1 h at RT with PE-anti-human IL-17A (0.5 μg ml −1 , clone 41802, R&D System). Stained cells were observed by fluorescence microscopy at ×40 magnifications using the Olympus BX51 upright microscope. Microarray analysis For microarray analysis, cultures of C. albicans SC5314 cells were grown in RPMI-1640 medium and treated with either 10 ng ml −1 IL-17A (R&D Systems) or drug vehicle, and incubated for 4 and 24 h at 37 °C. Total RNA was extracted with mortar and pestle in the presence of liquid nitrogen. The resulting powder was resuspended in TRIZOL (Invitrogen S.R.L., Milan, Italy) and transferred to a 1.5-ml Eppendorf tube, and gently vortexed and inverted two or three times to homogenize the sample. RNA was then amplified, biotin-labeled (MessageAmp II Biotin-Enhanced kit, Ambion Applied Biosystems, Monza, Italy) and purified on an affinity resin (RNeasy, Qiagen SpA, Milan, Italy). Hybridization was done automatically overnight (16 h) at 45 °C to Affymetrix yeast GeneChips according to the protocol in the Affymetrix GeneChip Expression Manual using Febit's RT Analyzer. Starting from raw data files, analysis was performed using both the Affymetrix MAS4 algorithm (at the service provider) and the PROP algorithm (at Cebit, Germany). Microarray data were generated from two biological replicates. Complementary DNA generated from cells exposed to drug vehicle alone was used as reference. Significantly modulated genes were selected from those whose expression was above twofold higher or lower than control samples (accession code GSE35153). Gene Ontology annotations Protein function was assigned using a standard set of Gene Ontology (GO) Slim biological process term sets available at the Candida Genome Database ( http://www.candidagenome.org ). Analysis of autophagy ATG8 localization by indirect immunofluorescence Localization of ATG8 in Candida SC5314 cells was assayed by indirect immunofluorescence using a rabbit polyclonal antibody against ATG8 (Abcam, Prodotti Gianni, Milan, Italy). Localization of ATG8 was performed on cells grown in RPMI-1640 supplemented with glutamine and 2% dextrose, and buffered with 0.165 M MOPS, pH 7. Cells (1×10 6 ml −1 ) were placed on microscope glass slides, incubated for 4 h at 37 °C for adhesion, and treated with 10 ng IL-17A or drug vehicle for additional 4 h at 37 °C. Nonspecific binding sites were blocked with PBS/BSA 2.5%. Slides were then sequentially incubated with Con A for 45 min at 37 °C, with 1:1,000 dilution of a rabbit polyclonal antibody to ATG8 in PBS/BSA 2.5% at 4 °C and finally with 1:50 dilution of anti-rabbit IgG secondary antibody conjugated to tetramethyl rhodamine isothiocyanate (TRITC) (Sigma Aldrich). Cells were visualized with a 40×0.75 magnification objective on the Olympus BX51 upright microscope. MDC labelling MDC labelling was performed on Candida SC5314 grown as above and placed on microscope glass slides in the presence of 1 and 10 ng ml −1 IL-17A. A stock solution of 25 mM MDC in ethanol–DMSO (1:1—vol:vol) was prepared. After 4 h, cells were stained with the fluorescent dye MDC (Sigma Aldrich) at a final concentration of 50 μM for 20 min in the dark. 4′-6-Diamino-2-phenylindole (DAPI, Molecular Probes, Invitrogen S.R.L.) was used to detect nuclei. After washing with water, cells were visualized with a 40×0.75 magnification objective on the Olympus BX51 upright microscope. Mice and infections Mice were housed in specific pathogen-free barrier facilities at the Animal Facility of Perugia University, Perugia, Italy and were used in accordance with protocols approved by the Animal Welfare Assurance A-3143-01. Female C57BL/6 mice, 8- to 10-week-old, were purchased from Charles River laboratories (Calco). Breeder pairs of IL-17A −/− and IL-17F −/− , generated as described [44] were kindly provided by Dr Burkhard Becher, University Hospital of Zurich, CH-8057 Zürich, Switzerland. For Candida infection, 10 8 cells of C. albicans wild-type SC5314 strain and its mutant strains atg9 Δ /atg9 Δ, the revertant atg9 Δ /atg9 Δ +ATG9 and TOR1-1/TOR1 , or the MKY 378 strain and the derived mutants, crh11 Δ and crh12 Δ were injected intragastrically. The infections with the two wild-type strains were similar, and the growth rate of the mutant strains was comparable to that of the corresponding wild-type strains in vitro (data not shown). For vaginal infection, estrogen-treated mice (0.1 mg of estradiol benzoate (Sigma Aldrich) in 0.1 ml oil subcutaneously every other day) were intravaginally inoculated with 5×10 4 stationary phase wild-type or crh11 Δ blastoconidia as described [45] . Two days post infection, lavage fluid cytospins were observed for fungal growth by light microscope, after May–Grünwald–Giemsa staining. For pulmonary aspergillosis, mice were anesthetized by intraperitoneal injection of 2.5% avertin (Sigma Chemical) before instillation of a suspension of 2×10 7 conidia per 20 μl saline intranasally of the Aspergillus AF293 wild-type and the crf1 Δ mutant strains. Cells were exposed to IL-17A (10 ng ml −1 ) or drug vehicle for 4 h at 37 °C in RPMI-1640 before injection. Mice were monitored for fungal growth and histology. Fungal growth was expressed as colony-forming units per organ, mean±s.e., obtained by serially diluting homogenates and plating them in triplicate on Sabouraud agar plates. For histology, paraffin-embedded tissue sections (3–4 μm) of stomach and lung tissues were stained with periodic acid-Schiff reagent. Photographs were taken using the Olympus BX51microscope. For SEM, the stomachs were removed at 2 days post infection and processed for SEM staining. Statistical analysis For multiple comparisons, P -values were calculated by using one-way analysis of variance (Bonferroni post-test), as specified for individual P -values described in figure legends. For single comparison, P -values were calculated by using two-tailed Student's t -test. The data reported are either from one representative experiment out of three to five independent experiments or are compiled from three to five experiments. At least six mice per group per experiment were used, as computed by power analysis to yield a power of at least 80% with an α -value of 0.05. Accession codes: Microarray data have been deposited in Gene Expression Omnibus under the accession code GSE35153 . How to cite this article: Zelante, T. et al . Sensing of mammalian IL-17A regulates fungal adaptation and virulence. Nat. Commun. 3:683 doi: 10.1038/ncomms1685 (2012).